Reversible patterning and actuation of hydrogels by electrically assisted ionoprinting The ability to pattern, structure, re-shape and actuate hydrogels is important for biomimetics, soft robotics, cell scaffolding and biomaterials. Here we introduce an ‘ionoprinting’ technique with the capability to topographically structure and actuate hydrated gels in two and three dimensions by locally patterning ions via their directed injection and complexation, assisted by electric fields. The ionic binding changes the local mechanical properties of the gel to induce relief patterns and, in some cases, evokes localized stress large enough to cause rapid folding. These ionoprinted patterns are stable for months, yet the ionoprinting process is fully reversible by immersing the gel in a chelator. The mechanically patterned hydrogels exhibit programmable temporal and spatial shape transitions, and serve as a basis for a new class of soft actuators that can gently manipulate objects both in air and in liquid solutions. The ability to control and programme the shape of soft materials, such as gels, can enable the development of artificial muscles [1] , [2] , micropatterned and shape-transforming sheets [3] , [4] , enviro intelligent sensors and actuators [5] , [6] , [7] , [8] , biomimetic microbots [9] , [10] , [11] , cell scaffolds [12] , [13] and drug delivery systems [14] , [15] . Hydrogels are networks of crosslinked hydrophilic polymers capable of absorbing and releasing large amounts of water while maintaining their structural integrity. They are a diverse class of soft, biocompatible materials composed of a tissue-like aqueous matrix with the capacity to change shape in response to external stimuli such as salinity [5] , pH [5] , [14] , temperature [6] , [16] , [17] or light [18] . The potential to locally pattern hydrogels with chemical or physical means can provide control over their physical response, which is useful in numerous applications such as soft actuators [5] , [6] , [7] , [8] , drug administers [14] , [15] , microvalves [19] and cell encapsulation [17] . Existing patterning techniques include, for example, moulding [15] , photolithography [14] , reaction-diffusion precipitation [3] and spatially varied crosslinking [20] . We believe that the ionoprinting, patterning and actuation method presented here is the first demonstration of electrical and directional embedding of ions within hydrated gel networks, locally crosslinking and mechanically stiffening the hydrogel. The use of electrical fields allows injecting an exact amount of ions, easily controlled by the duration and magnitude of the current. Electric field stimuli have been used to control the reaction-diffusion fronts of precipitating ions within gelatin [3] , [21] . Our method is distinguished by the use of electrochemically active electrodes to drive the diffusion and binding of ions to the ionic network of the hydrogel matrix. This reversible process can imprint topographic features in the hydrogel using modest voltages, tune its local mechanical properties to create physically reinforcing exoskeletons and generate stresses sufficient to actuate or fold hydrogels over large distances within seconds. In addition, the mechanical strain, coupled with the electrically directed binding and differential shrinkage, allows rapid and controllable actuation of the hydrogel with potential use in soft robotics. Principles of the ionoprinting technique The principles of ionoprinting are schematically shown in Fig. 1a ( Supplementary Movie 1 captures the process dynamics). Applying an oxidative bias to a flat or patterned metal anode (in this case, Cu) delivers ions to a polyelectrolyte (sodium polyacrylate; pNaAc) hydrogel as a result of the current through the gel. 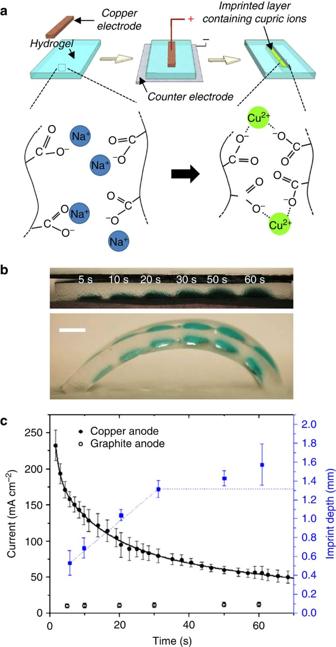Figure 1: Principles and example of the ionoprinting process. (a) By applying a potential to a patterned Cu anode, Cu2+ions complex locally with anionic hydrogels; (b) side view of an ionoprinted pNaAc gel using a 3.2-mm diameter copper cylinder at various time steps (5 V). The current determines the amount of copper bound to the hydrated network, which controls the depth of imprinting and degree of gel curvature as a result of ionic crosslinking. Scale bar=3 mm; (c) ionoprinting current and imprinted depth versus time based on triplicate experiments (5 V). The error bars represent s.d. The depth of the copper-imprinted layer was measured by micrographs of cross-sectional slices of the hydrogel. The superimposed blue line is only used to guide the eyes. Using inert graphite electrodes results in a background current of ~15 mA cm−2for the natural ionic conduction of the hydrogel. Figure 1: Principles and example of the ionoprinting process. ( a ) By applying a potential to a patterned Cu anode, Cu 2+ ions complex locally with anionic hydrogels; ( b ) side view of an ionoprinted pNaAc gel using a 3.2-mm diameter copper cylinder at various time steps (5 V). The current determines the amount of copper bound to the hydrated network, which controls the depth of imprinting and degree of gel curvature as a result of ionic crosslinking. Scale bar=3 mm; ( c ) ionoprinting current and imprinted depth versus time based on triplicate experiments (5 V). The error bars represent s.d. The depth of the copper-imprinted layer was measured by micrographs of cross-sectional slices of the hydrogel. The superimposed blue line is only used to guide the eyes. Using inert graphite electrodes results in a background current of ~15 mA cm − 2 for the natural ionic conduction of the hydrogel. Full size image The Cu 2+ ions generated at the anode/hydrated gel interface associate with the anionic carboxylic groups on the gel polymer backbone, forming robust localized ionic crosslinks in the gel network. The imprinted areas of the network release water due to the decrease in the hydration state of the polymer backbone, leading to a directed shrinking of the gel. The ionoprinting process results in a cyan-coloured embedded pattern containing copper metal ions with a relief structure that replicates the electrode mould on top of a translucent gel substrate ( Figs 1b and 2a ). These patterns of ions remain visibly stable for periods as long as months in a water bath. Electron paramagnetic resonance spectra from ionoprinted pNaAc hydrogels ( Supplementary Fig. S1 ) indicate that the cupric ions form monomeric complexes where one Cu 2+ ion binds to two carboxylic groups. As a result, two adjacent sodium counterions on the polymer backbone get displaced for a single cupric ion. The exact amounts of injected cupric ions have been confirmed experimentally using inductively coupled plasma optical emission spectroscopy (ICP-OES) (see Supplementary Fig. S2 for details). The strong electrostatic attraction between cupric ions and polysodium acrylate creates stable complexes with a binding constant of log ( β 102 ) ~6.6 (ref. 22 ), which is approximately 10 4 times larger than the complexes created by monomeric acid analogues [23] . 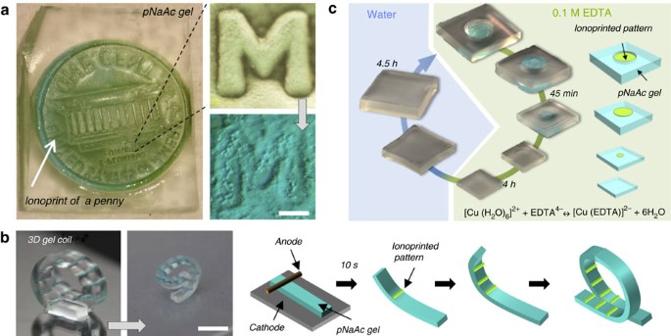Figure 2: Reversible 2D and 3D patterning by ionoprinting. (a) An ionoprinted pNaAc gel using a penny as the anode (15 s at 15 V). Features are replicated with high definition and can be scaled down by a factor of five after gel dehydration. Scale bar, 100 μm; (b) stresses induced by the lines ionoprinted with a (slightly tilted) copper wire anode are used to fold a 3D gel coil. This 3D shape is conserved when the gel is dehydrated. Scale bar, 5 mm. (c) a 3-mm-deep, 5-mm diameter circular pattern, ionoprinted on a pNaAc gel, is erased by immersion in EDTA for 4 h. The pattern disappears due to the chelation and the gel shrinks due to osmotic equilibrium in 0.1 M EDTA. The hydrogel sample was extracted from the solution to take the corresponding photos. Figure 2: Reversible 2D and 3D patterning by ionoprinting. ( a ) An ionoprinted pNaAc gel using a penny as the anode (15 s at 15 V). Features are replicated with high definition and can be scaled down by a factor of five after gel dehydration. Scale bar, 100 μm; ( b ) stresses induced by the lines ionoprinted with a (slightly tilted) copper wire anode are used to fold a 3D gel coil. This 3D shape is conserved when the gel is dehydrated. Scale bar, 5 mm. ( c ) a 3-mm-deep, 5-mm diameter circular pattern, ionoprinted on a pNaAc gel, is erased by immersion in EDTA for 4 h. The pattern disappears due to the chelation and the gel shrinks due to osmotic equilibrium in 0.1 M EDTA. The hydrogel sample was extracted from the solution to take the corresponding photos. Full size image The ionoprinting begins at voltages exceeding ~2–3 V, allowing a sufficient current to cross the gel and begin crosslinking the matrix (~30 mA cm −2 in the case of an applied potential of 5 V c.f. curve of Fig. 1c ). This threshold potential is in agreement with the sum of the activation potentials of the reactions occurring at each electrode–gel interface, oxidation of copper and reduction of hydrogen, and an overpotential that may exceed 1 V (ref. 24 ). Beyond this threshold potential, the initial electrophoretic mobility of Cu 2+ ions in the gel network (that is, determined from the slope of the curve on Fig. 1c ) is 1.1 × 10 −2 mm 2 V −1 s −1 . The cupric ions penetrate the gel until the relief-structured layer no longer has carboxylate groups available for binding, which subsequently passivates the ionic flow and leads to an imprint depth plateau ( Fig. 1c and Supplementary Fig. S2 ). The ionoprinting process is thus dependent on the composition of the hydrogel, that is, its content of charged carboxylate groups (see Supplementary Fig. S3 ). Consequently, the gel composition, the imprinting time or the applied voltage amplitude can be used to tune the depth of the ionoprinted patterns ( Fig. 1c and Supplementary Figs S3 and S4 ). Reversible high-fidelity ion crosslinking During the ionoprinting process, the localized complexation of copper generates stresses in the gel around the ionoprinting regions that can be harnessed for patterning and actuation. Figure 2a illustrates the high-fidelity replication of two-dimensional (2D) features such as those found on a penny. A structure or pattern can be robustly replicated with excellent spatial feature preservation. The resulting features in the gel are only 8–10% smaller laterally than the mould features due to predominant ion infusion in the direction normal to the electrode. The ionoprinting process enables hydrogels to be reversibly functionalized after polymerization and hydration. The replicated features can be further scaled down by a factor of five by drying the gel. The mechanical stresses developed during copper binding to the anionic network can be sufficient for rapidly folding 2D hydrogel slabs into three-dimensional (3D) shapes in air ( Figs 1b and 2b / Supplementary Movie 2 ). For a 3-mm-thick gel piece and an applied electric field of 5 V mm −1 the bending angle reaches 70° after 10 s. This rapid response results from the locally increased crosslinking density of the ionoprinted regions infused with copper ions. Finally, the structuring is fully reversible: immersing the gel in EDTA for ~4 h removes the cupric ions from the ionoprinted regions of the hydrogel network. This reversal is due to chelation, that is, complexation of cupric ions with the multidentate EDTA ligands. The removal of the Cu 2+ by the EDTA relieves the mechanical stresses, thereby restoring the original state of the gel. Upon rehydration (~30 min) the restored gel swells back to its initial non-ionoprinted state ( Fig. 2c ). Properties of ion patterns for differential swelling and shrinking In addition to providing new ways to pattern ions and topographically structure hydrogels, the ionoprinting process increases the stiffness of the hydrogel network due to ion chain crosslinking [25] . Flexible materials with stiff patterns have programmed directional folding and response as illustrated recently by Kumacheva et al. [4] and could find applications in actuators [6] or smart containers or capsules [26] . We hypothesized that the stiff ionoprinted regions of pNaAc gels could provide an exoskeleton dictating how the shape of the gel responds to stresses generated by contraction and expansion. We demonstrated the viability of this concept by making configurable shape memory soft materials and actuators such as grippers. The volume of ionic hydrogels can change readily under the action of stimuli such as temperature or pH; however, organic solvent-induced swelling and contraction offers a rapid and facile actuation that may not affect the binding of the complexed cupric ions. Thus, we patterned pNaAc hydrogels and placed them in an organic solvent medium (ethanol), which is known to evoke large and rapid shrinking of the native gel ( Supplementary Figs S5 and S6 ) [9] , [27] , [28] . The combined differential stiffness and shrinkage between the non-ionoprinted and ionoprinted regions are at the origin of the shaping mechanism, dictated by the geometrical design of the ionoprinting patterns. Various gel shapes are possible by ionoprinting on 3-mm thick hydrated samples. Initially, a U-shaped gel imprinted with five parallel lines bends upward and perpendicular to the patterned lines due to stresses induced by directed cupric ion complexation ( Fig. 3a ). After a few minutes in ethanol, the curvature of the gel inverts with the bending occurring along the direction of the imprinted lines. After 30 min of alcohol infusion, the gel adopts a cocoon-like shape because of the stronger deformation in the direction normal to the lines and a weaker deformation along their length. Overall, the whole gel structure shrinks asymmetrically adopting a shape dictated and preprogrammed by the ionoprinted exoskeleton. Placed back in water for 20 min, the gel recovers its original curved shape while transiently passing through a saddle-like transition configuration (with negative Gaussian curvature), probably resulting from the faster infusion with the new media from the sides of the slab. By controlling the orientation and spacing of the ionopatterned lines, one can create a variety of geometric responses. Importantly, intermediate gel structures preserve their shape after extraction from the solution. Thus, the ionoprinting technique enables a new class of solution-driven shape memory hydrogels: the ionoprinting preprogrammes the final gel shape, which is further controlled by the composition of the medium and time of immersion. These programmable soft materials illustrate a behaviour analogous to the ‘two-way’ memory effect [29] —the gel remembers the curvature induced by the ionoprinting process and can later be tuned to another curvature by solvent immersion. A gradient of curvature could be introduced by simply varying the amount of complexed ions ( c.f. Fig. 1b ), and more complex sequences to control the shape of ionic hydrogels both spatially and temporally in 2D and 3D can be designed. One example is given in Fig. 3b , where one region (labelled as i+) has been ionoprinted twice the time (10 s) compared to i− regions (see Supplementary Fig. S7 for further details). The ionoprinting patterns can also be used to embed 3D frameworks in the hydrogel to guide its shrinking and swelling ( Fig. 3c ). The ethanol/water cycles could be sustainably repeated for more than 10 times with only modest hysteresis, which may be caused due to insufficient time for thorough diffusion-driven replacement of the medium inside the gel ( Fig. 3d ). 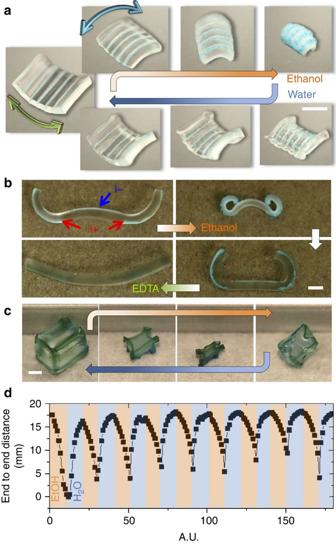Figure 3: Spatially and sequentially programmable 3D gel shapes. (a) 3-mm thick gel ionoprinted with five lines. As a result of the stresses developed during ionoprinting, the gel initially bends perpendicular to the imprinted directions (green arrow). Once immersed in EtOH (ethanol), the stiffer ionoprinted regions guide the asymmetric shrinking and reshaping of the gel structure (blue arrow). The initial shape recovers when placed in water. Scale bars, 15 and 10 mm, respectively; (b) example of a controlled shape by differential ionoprinting and subsequent time-dependent shape transformation after immersion in EtOH and EDTA, respectively. Scale bar, 5 mm. (c) a sequentially imprinted gel cube. The ionic crosslinks bind the imprints at the joints and provide a rigid frame controlling the structure during shrinking and swelling. Scale bar, 2 mm; (d) repetitive ethanol/water cycles of bending of a hydrogel strip imprinted with a single line, showing ~30% reduction in bending after ten cycles as measured by the end-to-end distance. Figure 3: Spatially and sequentially programmable 3D gel shapes. ( a ) 3-mm thick gel ionoprinted with five lines. As a result of the stresses developed during ionoprinting, the gel initially bends perpendicular to the imprinted directions (green arrow). Once immersed in EtOH (ethanol), the stiffer ionoprinted regions guide the asymmetric shrinking and reshaping of the gel structure (blue arrow). The initial shape recovers when placed in water. Scale bars, 15 and 10 mm, respectively; ( b ) example of a controlled shape by differential ionoprinting and subsequent time-dependent shape transformation after immersion in EtOH and EDTA, respectively. Scale bar, 5 mm. ( c ) a sequentially imprinted gel cube. The ionic crosslinks bind the imprints at the joints and provide a rigid frame controlling the structure during shrinking and swelling. Scale bar, 2 mm; ( d ) repetitive ethanol/water cycles of bending of a hydrogel strip imprinted with a single line, showing ~30% reduction in bending after ten cycles as measured by the end-to-end distance. Full size image To quantify the bending behaviour of the gel in ethanol, we characterized the impact of the width and thickness of the gel in a model slab ionoprinted structure depicted in the inset of Fig. 4a,b . Changing the gel width did not affect the bending capability of the gel, but delayed the onset of bending ( Fig. 4a ). However, thicker gels bend less than thinner gels ( Fig. 4b ). Gel dimensions can thus be adapted to precisely trigger and control their bending. The data for the curvature of the ionoprinted material as a function of thickness can be interpreted on the basis of Timoshenko’s model for metal bilayers [30] , [31] using a single fitting parameter (see Fig. 4c and Supplementary Fig. S8 for more details on the fitting model). 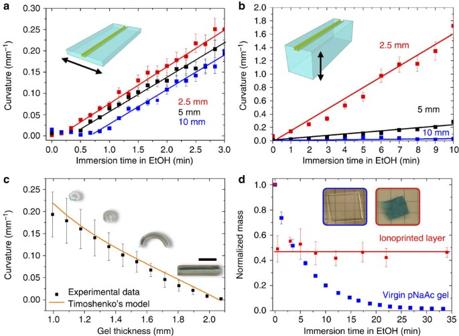Figure 4: Characterization of the bending behaviour of ionoprinted gel slabs in ethanol. (a) Bending curvature versus immersion time in EtOH (ethanol) for ionoprinted gels of various widths and a constant thickness of 3 mm. (b) bending curvature versus immersion time in EtOH for ionoprinted gels of various thickness and a constant width of 5 mm. (c) bending curvature as a function of the gel thickness. The simulation curve corresponds to Timoshenko’s model corrected with a fitting parameter of 0.5. Scale bar, 1 cm; (d) mass of a fully ionoprinted gel and a virgin one after immersion in EtOH. The amount of water rapidly expelled from the fully ionoprinted gel is compared with the virgin one. Inset gridlines are 5 mm apart. All of the above experiments were conducted in triplicate and error bars represent s.d. Figure 4: Characterization of the bending behaviour of ionoprinted gel slabs in ethanol. ( a ) Bending curvature versus immersion time in EtOH (ethanol) for ionoprinted gels of various widths and a constant thickness of 3 mm. ( b ) bending curvature versus immersion time in EtOH for ionoprinted gels of various thickness and a constant width of 5 mm. ( c ) bending curvature as a function of the gel thickness. The simulation curve corresponds to Timoshenko’s model corrected with a fitting parameter of 0.5. Scale bar, 1 cm; ( d ) mass of a fully ionoprinted gel and a virgin one after immersion in EtOH. The amount of water rapidly expelled from the fully ionoprinted gel is compared with the virgin one. Inset gridlines are 5 mm apart. All of the above experiments were conducted in triplicate and error bars represent s.d. Full size image The change in curvature of the patterned gel immersed in ethanol is caused by the asymmetric strain induced by the significantly different degrees of water expulsion from the native and ion-infused sections of the slabs combined with the differential shrinkage between those two regions. Figure 4d demonstrates that the expulsion of water from fully ionoprinted gels occurs much more rapidly than from virgin gels. The expulsion of water from the virgin gels is controlled initially by the mobility of the solvent molecules followed by shrinking due to relaxation of the polymer chains ( Supplementary Fig. S6 ). The Young’s moduli of the gels changes after ionoprinting and solvent exchange, which were measured to be 21, 300 and 66 kPa for virgin gels immersed in water, ionoprinted gels and ethanol, respectively ( Supplementary Material , including Supplementary Figs S5 and S6 ). Ionoprinting for soft matter actuation The ionoprinting technique enables a proof-of-principle demonstration of two distinct classes of soft actuators capable of gently and precisely manipulating lightweight objects (0.1–1 g ) with a fast response. The first proposed mechanism of gel actuation is based on the stress generated by ionoprinting in air ( Supplementary Movie 2 ). We realized a prototype of soft tweezers by placing a Λ-shaped gel in contact with two copper wires, (C1) and (C2). Applying a positive potential to the inner C1 electrode generates an ionoprinted line near the vertex. The ionic injection produces enough directed stress to close the Λ-gel on itself and grab the object. Reversing the potential folds the gel in the opposite direction, opening the tweezers and releasing the object ( Fig. 5a , Supplementary Movie 3 ). Repetitive use of such kind of actuators are limited to 2–3 cycles as the gel saturates with copper ions ( c.f. Fig. 1c ). Immersion in EDTA solution and subsequently in water rejuvenates the actuator. The second actuation mechanism uses the shape memory effect described in Fig. 3 and operates in liquid medium. 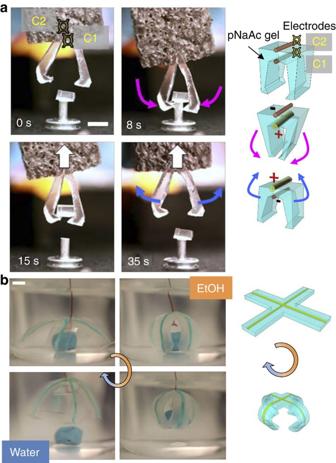Figure 5: Prototypes of soft actuators. (a) The stress induced by an applied potential folds the gel towards the anode. By alternating the field, the soft tweezers can handle and release a 0.1-g polydimethylsiloxane cube. Scale bar, 10 mm; (b) an X-shaped gel suspended with a wire permits extraction of a small 1 g blue cube of polydimethylsiloxane from ethanol solution and its subsequent release in water. Scale bar, 10 mm. Figure 5b illustrates a prototype of soft tweezers functioning based on this principle. It consists of an X-shaped gel ionoprinted with two perpendicular lines along one side of its appendages. The expulsion of water drives the gel folding in ethanol to a create uniform curvature along the ionoprinted lines, which gently grips small objects. Placing the gel tweezers back in water causes the gel network to rehydrate and return to its initial state, while releasing the enclosed object in the process ( Fig. 5b and Supplementary Movie 4 ). Figure 5: Prototypes of soft actuators. ( a ) The stress induced by an applied potential folds the gel towards the anode. By alternating the field, the soft tweezers can handle and release a 0.1-g polydimethylsiloxane cube. Scale bar, 10 mm; ( b ) an X-shaped gel suspended with a wire permits extraction of a small 1 g blue cube of polydimethylsiloxane from ethanol solution and its subsequent release in water. Scale bar, 10 mm. Full size image We introduce ionoprinting as a facile and rapid technique to reversibly pattern ions in hydrogels in 2D and 3D by directionally controlled injection and binding of ions. The ionoprinted gel regions exhibit an order of magnitude larger modulus than the virgin ones, and thus have been used as exoskeletons to guide anisotropic actuation of gel structures under volumetric changes once placed in an organic solvent. As the ionoprinting process can be extended to other biocompatible divalent ions such as Ca 2+ or Zn 2+ ( Supplementary Fig. S9 ), we believe that this technique can find applications in drug delivery, ion-mediated chemistry and in the fabrication of scaffolds with spatial control of ion concentration for tissue engineering. The ionoprinting process can also be employed easily to design and programme soft material actuators. We apply this technique to create soft tweezers working independently in air and in liquid solution. These simple examples point out the potential application of similar gel actuators in the precise manipulation of small objects in various environments and in future biomimetic soft robots. Materials Anhydrous acrylic acid 99% (AA, Sigma, Lot# SHBB0493V), acrylamide (AAm, Sigma, Lot# 021M0170V), N , N ′-methylenebis(acrylamide) (Sigma, Lot# 120M0109V), ammonium persulfate (APS, Sigma, Lot# 047K2503V), N , N , N ′ N ′-tetramethylethylenediamine 99.5% (TEMED, Sigma, Lot# 10588KD), Agarose LE (Acros Organics, Lot# A0268063), calcium chloride dihydrate (Sigma, Lot# 09108LE), sodium hydroxide (Acros Chemical, Lot# A017823701) and EDTA(Sigma, Lot# 031M8709) were used as received. Sodium acrylate was prepared in situ by adding equimolar amounts of acrylic acid and sodium hydroxide to the precursor mixture. The gels were prepared and equilibrated in Milli-Q deionized water (18.2 MΩ cm). Copper wire (0.5 mm) was used from Alfa Aesar (Lot3 L15T005) and the copper pellets 99.99% were from Kurt Lesker (l/4′ Lot# CU1049749091 and 1/8′ Lot# CU10149750401). Hydrogel fabrication Poly(sodium acrylate) hydrogel was prepared by free-radical polymerization in aqueous solution using N , N ′-methylenebis(acrylamide) as the crosslinker. APS and TEMED were used as the initiator and accelerator, respectively. The overall monomer concentration was fixed at 5 M and the crosslinker ratio (mole ratio of divinyl to vinyl monomers) was fixed at 1:200. The monomers were dissolved along with 67 μl of APS in 5 ml of water. After addition of 25 μl of TEMED, 1.2 ml of solution was injected between two glass slides separated by a 1-mm-thick silicon spacer. The hydrogel sheets were removed from a 70 °C oven after 3 h and placed in an excess of Milli-Q water for at least 24 h before experimentation. Ionoprinting technique Cupric ions were patterned into the gel network by superficially drying the pNaAc gel, then placing it in contact with a copper (anode) and aluminium (cathode) electrode and applying the desired potential. The current through the gel was characterized using a Keithley 2410 Sourcemeter with Lab Tracer 2.0 software. EPR experiments X-band electron paramagnetic resonance (EPR) spectra of imprinted samples for various imprinting times were recorded at room temperature using a Bruker Biospin (Billerica, MA) Elexsys 580 spectrometer. The experimental parameters were as follows: microwave frequency ν ~9.870 GHz, incident microwave power=2 mW, modulation amplitude=5 G, modulation frequency=100 kHz and time constant=10.24 ms. ICP-OES measurements After the ionoprinting process, the gel samples were immersed in 0.1 M EDTA solutions for 2 weeks. Samples were analysed for copper concentration using ICP-OES, which was performed using a Perkin Elmer 2000 DV ICP-OES utilizing a cross-flow nebulizer with the following parameters: plasma 18.0 l Ar (g) min −1 ; auxiliary 0.3 l Ar (g) min −1 ; nebulizer 0.73 l Ar (g) min −1 ; power 1,500 W; peristaltic pump rate 1.40 ml min −1 . Instrument reproducibility ( n =10) determined using 1 mg l −1 elemental solutions resulted in <±2% error. How to cite this article: Palleau, E. et al. Reversible patterning and actuation of hydrogels by electrically assisted ionoprinting. Nat. Commun. 4:2257 doi: 10.1038/ncomms3257 (2013).